Implementation of generalized quantum measurements for unambiguous discrimination of multiple non-orthogonal coherent states Generalized quantum measurements implemented to allow for measurement outcomes termed inconclusive can perform perfect discrimination of non-orthogonal states, a task which is impossible using only measurements with definitive outcomes. Here we demonstrate such generalized quantum measurements for unambiguous discrimination of four non-orthogonal coherent states and obtain their quantum mechanical description, the positive-operator valued measure. For practical realizations of this positive-operator valued measure, where noise and realistic imperfections prevent perfect unambiguous discrimination, we show that our experimental implementation outperforms any ideal standard-quantum-limited measurement performing the same non-ideal unambiguous state discrimination task for coherent states with low mean photon numbers. Measurement of the quantum properties of a physical system is fundamental in quantum mechanics and quantum information science [1] , [2] , [3] , [4] . Quantum mechanics prohibits the perfect discrimination of non-orthogonal states due to their intrinsic overlap. This seemingly impossible task can, however, be accomplished by performing generalized quantum measurements that allow for inconclusive results as a possibility for the measurement outcomes. Quantum-state discrimination among non-orthogonal states, besides being of fundamental interest, is critical for many realizations of quantum information processing. In particular, the discrimination of non-orthogonal coherent states is essential in quantum key distribution for unconditionally secure communications [5] , [6] , [7] , [8] and coherent-state-based quantum repeaters [9] , [10] and quantum computing [11] , [12] , [13] . Moreover, multi-state discrimination can enable coherent-state-assisted entanglement generation with high fidelity [14] , entanglement swapping [15] and photon number state preparation and detection [11] . In addition, unambiguous multi-state comparison allows for quantum digital signatures [16] . There are two complementary approaches for non-orthogonal state discrimination. The first of these, minimum error discrimination (MED), seeks measurements that minimize the probability of erroneously identifying the state [2] . The second approach, unambiguous state discrimination (USD), introduces inconclusive results to achieve perfect state discrimination [17] , [18] , [19] and aims to maximize the probability of conclusive results. However, imperfections in realistic implementations make ideal (error-free) USD impossible. Thus, real-world USD becomes an intermediate measurement strategy between MED and ideal USD, which retains the conclusive results of ideal USD, but contains some errors in those conclusive results. Although there do exist post-selection-based conventional measurement techniques for coherent states characterized by errors and inconclusive results, they cannot improve upon standard-quantum-limited performance [2] , [20] , [21] . Thus, the goal becomes to realize a USD measurement with realistic imperfect devices that does surpass this conventional measurement limit. In contrast to significant efforts in MED [2] , [22] , [23] , [24] , [25] , [26] , [27] , [28] , studies of USD of non-orthogonal coherent states have been limited [21] , [29] , [30] , [31] , and experiments have been restricted to discrimination of just two coherent states [32] . Moreover, the feasibility of implementing a USD measurement for multiple non-orthogonal coherent states, and whether implementation in the presence of imperfections can outperform any ideal standard-quantum-limited measurement, has been an open question. An analogous effort to demonstrate the superiority of USD implementations for multiple qubits, but over optimal projective measurements, was attempted in ref. 33 , but without success [34] . Recently, the implementation of generalized measurements for optimal USD of two matter qubits was demonstrated and shown to outperform the standard ideal projective measurements [35] . We demonstrate the first realization of generalized quantum measurements for USD of four non-orthogonal coherent states using coherent displacement and photon counting. We present a full quantum mechanical description of this USD measurement in the form of a positive-operator valued measure (POVM), and we derive the probabilities of conclusive results and the corresponding errors resulting from imperfections of the real experimental implementation. We show that our USD implementation, even though it uses a suboptimal strategy, which does not maximize the probability of conclusive results, outperforms the ideal conventional standard-quantum-limited measurement for the discrimination of four non-orthogonal coherent states at low mean photon numbers. In addition, our USD implementation is scalable to higher numbers of coherent states, and should be applicable to future implementations of quantum information processing and quantum measurements. POVMs for USD of multiple coherent states USD of non-orthogonal states is possible with a measurement process that allows for what are termed inconclusive results. As a result, the number of outcome possibilities of the USD measurement process is one greater than the number of possible states of the system under test. Generalized quantum measurements for USD of four non-orthogonal symmetric coherent states, , with equal initial probabilities, , ( k =1,..,4), are described by a complete set of POVMs, , m =1,…,5 satisfying and for all m (ref. 36 ). The outcomes of the measurement operators unambiguously identify one of the possible non-orthogonal states, and corresponds to an inconclusive result. The probability of obtaining an inconclusive result is , where is the probability of an inconclusive result given the input state . There is a known theoretical optimal solution for USD of linearly independent symmetric non-orthogonal states, which maximizes the probability of conclusive results, p conc =1− p inc (ref. 36 ). In particular, there is a known scheme, which, in the limit of small amplitudes, approaches optimality for multiple coherent states based on feed forward and photon counting [30] . However, finding a USD strategy which is optimal for any input powers for these states is an open problem. Here we implement a measurement scheme for suboptimal USD for four non-orthogonal states based on displacement operations and photon counting [30] (see Fig. 1a ). 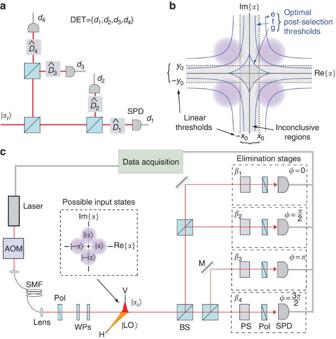Figure 1: Non-orthogonal unambiguous multi-state discrimination. (a) Scheme for USD of four non-orthogonal coherent states. (b) Ideal standard-quantum-limited measurement with an inconclusive region, enclosed by linear thresholds defined byx0andy0(black dashed lines) where (x,y)=(Re{α}, Im{α}), can perform an intermediate discrimination measurement analogous to a non-ideal USD measurement. Alternatively, the optimal post-selection thresholds e, f and g (solid blue lines) define the optimal regions resulting in the lowest probability of error for three examples of different conclusive result probabilities 0.34 (e), 0.65 (f) and 0.93 (g) for a fixed mean photon number of 1. This scheme decreases the probability of error by increasing the region for inconclusive results defined either by the linear post-selection thresholdsx0andy0, or by the optimal post-selection thresholds, which result in the lowest probability of error. (c) Experimental implementation of POVM for USD of four non-orthogonal coherent states. The inset shows the four non-orthogonal symmetric coherent states under measurementwith phasesφ={0,π/2,π, 3π/2}. AOM, acousto-optic modulator for pulse preparation; WPs, waveplates for state preparation; SMF, single-mode fibre;state under measurement with vertical (V) polarization;, auxiliary displacement field with horizontal (H) polarization; BS, 50/50 non-polarizing beam splitter; PS, phase shifter; Pol, polarizer; SPD, single-photon detector; M, mirror. Figure 1: Non-orthogonal unambiguous multi-state discrimination. ( a ) Scheme for USD of four non-orthogonal coherent states. ( b ) Ideal standard-quantum-limited measurement with an inconclusive region, enclosed by linear thresholds defined by x 0 and y 0 (black dashed lines) where ( x , y )=(Re{ α }, Im{ α }), can perform an intermediate discrimination measurement analogous to a non-ideal USD measurement. Alternatively, the optimal post-selection thresholds e, f and g (solid blue lines) define the optimal regions resulting in the lowest probability of error for three examples of different conclusive result probabilities 0.34 (e), 0.65 (f) and 0.93 (g) for a fixed mean photon number of 1. This scheme decreases the probability of error by increasing the region for inconclusive results defined either by the linear post-selection thresholds x 0 and y 0 , or by the optimal post-selection thresholds, which result in the lowest probability of error. ( c ) Experimental implementation of POVM for USD of four non-orthogonal coherent states. The inset shows the four non-orthogonal symmetric coherent states under measurement with phases φ ={0, π /2, π , 3 π /2}. AOM, acousto-optic modulator for pulse preparation; WPs, waveplates for state preparation; SMF, single-mode fibre; state under measurement with vertical (V) polarization; , auxiliary displacement field with horizontal (H) polarization; BS, 50/50 non-polarizing beam splitter; PS, phase shifter; Pol, polarizer; SPD, single-photon detector; M, mirror. Full size image The unknown state enters a branched set of beam splitters with four outputs . Each output undergoes a coherent displacement so that → with , and a single-photon detector (SPD) detects the photons in the displaced state with two outcomes d i ={0,≠0} representing the absence or presence of photons, respectively. A photon detection d i ≠0 in one of the ports unambiguously eliminates one possibility for the input state . Thus, by performing joint detections in the four ports, the four-element joint-detection event DET={ d 1 , d 2 , d 3 , d 4 } with one null detection in detector j , d j =0, and non-zero photon detections in all the other detectors, d i ≠0 ( i ≠ j ), unambiguously identifies the input state as . The POVM describing the USD operations realized in this scheme is a generalization of the optimal USD of two coherent states [29] and can be expressed as: for i =1,2,3,4, where with â and â † being the creation and annihilation bosonic operators, respectively, and β i the displacements of the input field. and and the symbol :: means normal ordering where indicates evaluation of operator under the constraint ( a < b < c …). These operators, covering all possible combinations of states, are related to the joint projection operations of the input state onto different test states performed by the USD measurement. The measurement operator describing an inconclusive result measurement is . In the presence of imperfections of realistic implementations, the probability of conclusive results is obtained from and is given by: where G k =1− F k , and . quantifies the mode mismatch between the input state and displacement field and is defined as , where is the measured visibility of the displacement operation, and η is the system detection efficiency. The first term in equation (2) is the contribution from correct identifications, , and the second term comes from erroneous identifications, ( i ≠ k ). The probability of error given the probability of conclusive results is ( j ≠ k ). 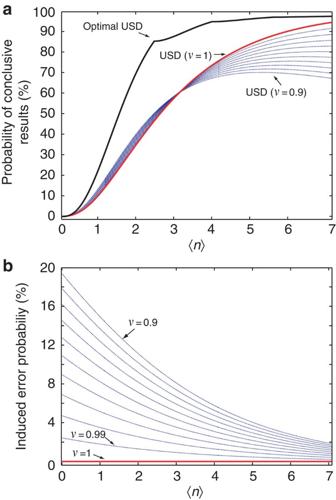Figure 2: Theoretical probability of conclusive results and errors. (a) Probability of conclusive results as a function of mean photon numberfor the USD scheme with different values of mode-mismatch visibility from(solid red line) toin steps of 0.01 (dotted lines) with 100% detection efficiency. For reference, the solid black line shows the theoretical maximum probability of conclusive results for the optimal USD36(b) Probability of errors for the USD scheme with the same mode-mismatch visibilities as panela. For this realization, the probability of error is Figure 2 shows the probability of conclusive results, and the probability of errors, as a function of mean photon number of the input state for the USD scheme [30] of Fig. 1a , with 100% detection efficiency and visibilities ranging from 0.9 to 1. The maximum probability of conclusive results for optimum USD is included in Fig. 2a as a reference from ref. 36 . For small mean photon numbers, the probability of conclusive results increases slightly as the visibility decreases from owing to an increase of the probability of photon detections caused by imperfections in the system. At the same time, the probability of errors increases rapidly as degrades in this few-photon-number region. The decrease in the probability of conclusive results at high mean photon numbers, as degrades, results from the possibility of non-zero photon detections due to the leakage, even when no photon should be seen. Figure 2: Theoretical probability of conclusive results and errors. ( a ) Probability of conclusive results as a function of mean photon number for the USD scheme with different values of mode-mismatch visibility from (solid red line) to in steps of 0.01 (dotted lines) with 100% detection efficiency. For reference, the solid black line shows the theoretical maximum probability of conclusive results for the optimal USD [36] ( b ) Probability of errors for the USD scheme with the same mode-mismatch visibilities as panel a . Full size image An intermediate measurement between MED and USD containing errors and conclusive events, analogous to the non-ideal USD process in realistic implementations of this POVM for USD, can be performed by an ideal standard-quantum-limited measurement corresponding to the heterodyne measurement with conclusive postselection [2] , [21] . The measurement operators describing conclusive results for the ideal heterodyne measurement are , where Г i defines the post-selection region in phase space. Figure 1b shows examples of the ideal heterodyne measurement with different post-selection regions Г i delimited by either the linear post-selection thresholds x 0 and y 0 (dashed lines), or by the optimal post-selection thresholds indicated with blue lines, which result in the lowest error for a given probability of conclusive results. This measurement can decrease the probability of error by increasing the region for inconclusive results with different post-selection thresholds. (The states under measurement shown in Fig. 1b have been rotated by π /4 compared with the states in our implementation for clarity, and to simplify the calculations without loss of generality.) The probability of conclusive results using linear post-selection thresholds x 0 and y 0 for the input state as a function of threshold x 0 = y 0 is and the probability of error for these post-selected results is The optimal post-selection regions for this intermediate measurement regime with errors and inconclusive results are found using numerical methods analogous to the work in ref. 37 . These optimal post-selection regions result in the same probability of conclusive results as the realistic implementation of USD under the constraint that each region contains events with the lowest probability of error for a given input state with a fixed mean photon number (see Methods). In this way, these optimal post-selection regions ensure the lowest probability of errors for a given probability of conclusive results. Therefore, it is possible to compare the performance of any realistic implementation of the POVM for USD, performing a non-ideal USD process to the ideal standard-quantum-limited measurement by investigating the error probabilities of both schemes for a fixed probability of conclusive results [20] . Experimental realization of multi-state USD We implement the POVM for USD of four non-orthogonal coherent states, investigate the discrimination process in realistic experimental conditions, and compare its performance with ideal standard-quantum-limited measurements implementing an intermediate discrimination process [2] , [20] , [21] . Figure 1c shows our experimental implementation of generalized quantum measurements for USD of four non-orthogonal symmetric coherent states with equal input probabilities. An acousto-optic modulator and a set of waveplates prepare the state under measurement and the auxiliary displacement field in the two orthogonal polarization modes of 100 ns light pulses [27] at a rate of 40 kHz. The mean photon number of the input state varies from 0.1 to 3, and the displacement field is 100 times stronger than the input state. These fields enter a set of three branched beam splitters, and the four outputs are directed to four elimination stages. Each stage is set to eliminate a given possibility for the phase φ ={0, π /2, π , 3 π /2} of the input state by displacement of this state and photon counting. The displacement operation is performed with a phase shifter that controls the relative phases of the input and auxiliary fields, and a projection onto a given polarization axis with a polarizer. This axis is chosen to transmit 99% of the input field and 1% of the strong auxiliary field so that after this projection both fields have equal strengths [27] . When the relative phase between these fields is π , this projection displaces the input field to the vacuum. An SPD in each elimination stage detects the presence or absence of photons in the displaced state, allowing for the elimination of a possible phase of the incoming state. The measured efficiencies of the SPDs are 84.0(5), 84.0(5), 83.0(5) and 82.0(5)%, and with 15 dark counts per second, which has a negligible effect on the USD measurement (all uncertainties quoted in this paper represent 1 s.d., combined statistical and systematic uncertainties). The total detection efficiency of the system is 75(1)%, which corresponds to the average of the efficiencies of the four elimination stages, which are 80.0(5), 78.0(5), 70.8(5) and 70.5(5)%, and account for the optical losses in each stage and the detection efficiency of the SPDs. The losses in each stage account for the splitting losses of the BSs and mirrors, and the optical components inside the stages that perform the displacement operations and couple light into the SPDs. The measured average visibility is % limited by amplitude and phase mismatch and all other imperfections. The joint detection events DET={ d 1 , d 2 , d 3 , d 4 } of the SPDs in the elimination stages with only one null result correspond to conclusive measurements of the POVM in equation (1). The probability of conclusive results correspond to the ratio of the number of observed conclusive events to the total number of experimental trials, which ideally correspond to a perfect USD. Any other case of joint photon detection events correspond to inconclusive results. The probability of error caused by reduced visibility corresponds to the ratio of the number of errors to the number of conclusive results. 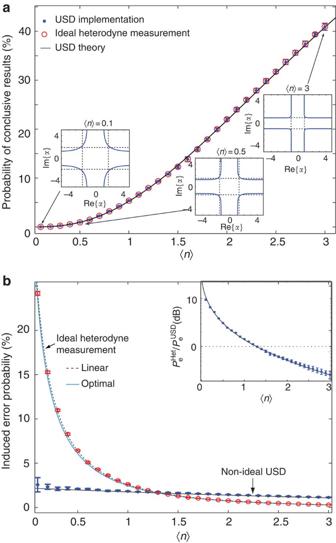Figure 3: Experimental probability of conclusive results and errors. (a) Experimental conclusive results as a function of mean photon number (blue dots), the theoretical predictions for the experimental parameters (solid black line) and for the ideal heterodyne measurement with adjusted linear thresholds (x0,y0) where (x,y)=(Re{α}, Im{α}), or with an optimal post-selection region (open red circles), to obtain the same probability of conclusive results as the implementation of non-ideal USD. Insets show the linear post-selection thresholds (dashed lines) and optimal thresholds (solid lines) for mean photon numbers 0.1, 0.5 and 3. (b) Experimental probability of error (blue dots), theoretical predictions of non-ideal USD for the experimental parameters (solid black line) and the probability of error of the ideal heterodyne measurement for the same probability of conclusive results with linear post-selection thresholds (open circles) together with the theoretical prediction (black dashed line). The lowest probability of error obtained with heterodyne measurement using optimal post-selection regions is shown with a solid blue line. Inset shows the ratio of the probability of errorsin dB. The error bars represent 1−σ statistical uncertainties. Figure 3a shows the measured probability of conclusive results as a function of mean photon number together with the theoretical predictions from equation (2), incorporating the experimental detection efficiency and visibility. The experimental data points result from four independent sets, each consisting of 10 6 independent experiments, and the error bars represent 1−σ statistical uncertainty. Figure 3b shows the errors by mode mismatch for the experimentally conclusive results together with the theoretical predictions from equation (3) for the measured experimental parameters. We observe an excellent agreement between the experimental observations and the theoretical predictions for the measured detection efficiency and visibility. Figure 3: Experimental probability of conclusive results and errors. ( a ) Experimental conclusive results as a function of mean photon number (blue dots), the theoretical predictions for the experimental parameters (solid black line) and for the ideal heterodyne measurement with adjusted linear thresholds ( x 0 , y 0 ) where ( x , y )=(Re{ α }, Im{ α }), or with an optimal post-selection region (open red circles), to obtain the same probability of conclusive results as the implementation of non-ideal USD. Insets show the linear post-selection thresholds (dashed lines) and optimal thresholds (solid lines) for mean photon numbers 0.1, 0.5 and 3. ( b ) Experimental probability of error (blue dots), theoretical predictions of non-ideal USD for the experimental parameters (solid black line) and the probability of error of the ideal heterodyne measurement for the same probability of conclusive results with linear post-selection thresholds (open circles) together with the theoretical prediction (black dashed line). The lowest probability of error obtained with heterodyne measurement using optimal post-selection regions is shown with a solid blue line. Inset shows the ratio of the probability of errors in dB. The error bars represent 1−σ statistical uncertainties. Full size image We evaluate the advantage of our realization of the POVM for USD of four non-orthogonal states over the ideal standard-quantum-limited measurement. We observe that our POVM implementation for USD (shown in Fig. 1c ) achieves lower error probabilities than the ideal standard-quantum-limited measurement for small mean photon numbers at a given probability of conclusive results. Figure 3a shows the probability of conclusive results for the ideal heterodyne measurement, where we have adjusted the linear post-selection threshold x 0 in equation (4), or alternatively applied optimal post-selection thresholds, to obtain the same conclusive result probabilities as in the experimental USD implementation. The insets show examples of the linear and optimal thresholds for mean photon numbers of 0.1, 0.5 and 3. We observe that for our experimental conclusive results and mean photon numbers, the heterodyne measurements with linear thresholds and optimal thresholds result in similar post-selection regions. The corresponding error probabilities of the ideal heterodyne measurement with linear thresholds, for these values of the probabilities of conclusive results, are shown in Fig. 3b (red open circles) together with the theoretical predictions from equation (5) (dashed black line), and for the heterodyne measurement with optimal postselection (solid blue line). Note that this corresponds to a perfect ideal heterodyne measurement with perfect detection efficiency and that, for the experimental parameters, optimal postselection shows only slightly lower errors than heterodyne with linear post-selection thresholds. We observe that our USD implementation performs with much lower errors, up to nine times lower, than is achievable with ideal standard-quantum-limited measurements for mean photon numbers up to 1, without any adjustment for system detection efficiency. These results highlight the real advantage of our USD implementation over ideal conventional technologies performing the same non-ideal USD process. In conclusion, the realization of generalized quantum measurements is essential for many quantum information and quantum metrology applications. We have demonstrated the first experimental realization of a POVM for USD of multiple non-orthogonal coherent states. Given the unavoidable noise and imperfections in any realistic implementation of these generalized measurements, we showed that our USD implementation outperforms any ideal standard-quantum-limited measurement for small mean photon numbers. Furthermore, because of its simplicity, the experimental scheme is scalable to higher numbers of coherent states. This implementation represents an important advance in state discrimination and quantum measurements, and can be applied to many quantum information tasks based on coherent states with small mean photon numbers. Optimal post-selection regions For a set of input states with prior probabilities { p i }, the heterodyne measurement with an optimal choice of post-selection region gives a probability of conclusive results where , and is the measurement operator density in quadrant j in the phase space with ( x , y )=(Re{ α }, {Im{ α }). Here R b ( x , y ) is the optimal post-selection region consisting of points ( x , y ) satisfying , where is the conditional error probability for point ( x , y ) and b is the maximum value of conditional error probability for points in R b . Thus, R b contains only points in phase space with the probability of conditional error lower than or equal to b , and minimizes the conditional error probability for a certain probability of conclusive results given by equation (6). We find the optimal postselection region resulting in the same probability of conclusive results as our USD implementation by numerically solving the equation In this way, R b ( x , y ) defines a post-selection region with the minimum probability of error for a given probability of conclusive results equal to our USD implementation. This is analogous to the optimization process in ref. 37 to find the post-selection area in phase space for maximizing the mutual information [38] . How to cite this article: Becerra F. E., et al. Implementation of generalized quantum measurements for unambiguous discrimination of multiple non-orthogonal coherent states. Nat. Commun. 4:2028 doi: 10.1038/ncomms3028 (2013).